Measuring long-range carrier diffusion across multiple grains in polycrystalline semiconductors by photoluminescence imaging Thin-film polycrystalline semiconductors are currently at the forefront of inexpensive large-area solar cell and integrated circuit technologies because of their reduced processing and substrate selection constraints. Understanding the extent to which structural and electronic defects influence carrier transport in these materials is critical to controlling the optoelectronic properties, yet many measurement techniques are only capable of indirectly probing their effects. Here we apply a novel photoluminescence imaging technique to directly observe the low temperature diffusion of photocarriers through and across defect states in polycrystalline CdTe thin films. Our measurements show that an inhomogeneous distribution of localized defect states mediates long-range hole transport across multiple grain boundaries to locations exceeding 10 μm from the point of photogeneration. These results provide new insight into the key role deep trap states have in low temperature carrier transport in polycrystalline CdTe by revealing their propensity to act as networks for hopping conduction. The inherent presence of defect states in semiconductors invariably influences carrier transport, yet the degree to which they affect electrical behaviour is determined by the nature of the defect and the properties of the semiconductor host. Polycrystalline CdTe (poly-CdTe) provides an interesting and important case study for exploring the interaction of carriers with defect states because it contains a rich admixture of electrically active and inactive defects. Further, some of these electrically active defects appear to be relatively benign. For example, poly-CdTe solar cells have demonstrated photovoltaic conversion efficiencies as high as 18% despite grain sizes of only a few microns in diameter [1] . The performance of the device is enhanced partially through the intentional and unintentional introduction of impurities (that is, O, Cl and Cu), which are thought to improve charge transport by altering the grain structure, the electrostatic potential barriers at grain boundaries and the electrical activity of grain boundary defect states [2] , [3] , [4] . These impurities also form deep trap states throughout the bulk material [5] , [6] . Establishing a detailed and accurate account of the relationship between grain boundaries, impurities and carrier transport in polycrystalline semiconductors requires a direct method of probing carrier diffusion paths. Here we present an investigation of carrier diffusion through poly-CdTe using a novel photoluminescence (PL) imaging technique. Our results reveal that the grain boundaries in this material are relatively transparent to exciton diffusion and that a network of deep acceptor states can actually assist hole transport over long distances at low temperatures (~80 K). The identification of preferential pathways for carrier transport and direct correlation with the microstructure and impurity distribution provides greater insight into the electrical properties of polycrystalline materials. PL imaging technique We use a new PL imaging technique to observe the extent to which carriers diffuse from a singular point of photogeneration. The general concept of the approach is shown in Fig. 1 . A laser beam is focused to a 1-μm spot incident on the sample ( Fig. 1a ). PL produced by radiative recombination of the photoinjected carriers is simultaneously collected by an objective lens over a large area of the sample and is projected onto a Si charge-coupled device (CCD) camera ( Fig. 1b ). Thus, PL is accurately mapped to the location of carrier recombination rather than the point of photogeneration, and an image of the spatial distribution of PL surrounding the point of photocarrier injection is generated instantaneously without scanning ( Fig. 1c ). Conventional cathodoluminecence and electron beam-induced current techniques, on the other hand, assign all carrier recombination or collection to the point at which they were generated, which does not preserve spatial diffusion information [7] , [8] . Decoupling the carrier generation and PL collection mechanisms in the present technique therefore has the advantage that it yields a true indication of how far carriers have diffused before they recombine. Observation of PL from a grain adjacent to one in which carriers are photoinjected provides unambiguous evidence that carriers have diffused across the grain boundary. A discontinuous change in the PL intensity from one grain to the next, as depicted in the schematic illustration in Fig. 1c , would otherwise suggest that carriers are at least partially blocked from diffusing across the grain boundary. Finally, a key feature of this technique is that it uses a tunable liquid crystal filter, placed between the objective lens and CCD camera, to detect only within narrow wavelength ranges (5–10 nm) such that PL from defect states can be imaged independently from band edge luminescence. This feature permits the observation of defect-mediated carrier diffusion. 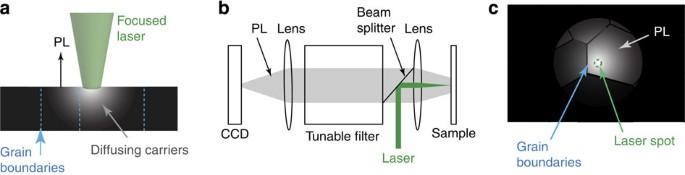Figure 1: Schematic of PL imaging measurement approach. (a) Cross-sectional view. Carriers are photogenerated in a single grain with a focused laser beam. (b) Beam path of experimental set-up. The resulting PL excited with a focused laser beam is collected from a large area of the sample with an objective lens and is imaged onto a Si CCD camera. (c) An illustrative schematic of a PL image showing how carrier interaction with grain boundaries might affect the PL intensity in adjacent grains. Figure 1: Schematic of PL imaging measurement approach. ( a ) Cross-sectional view. Carriers are photogenerated in a single grain with a focused laser beam. ( b ) Beam path of experimental set-up. The resulting PL excited with a focused laser beam is collected from a large area of the sample with an objective lens and is imaged onto a Si CCD camera. ( c ) An illustrative schematic of a PL image showing how carrier interaction with grain boundaries might affect the PL intensity in adjacent grains. Full size image PL of poly-CdTe The time-integrated PL spectrum of a CdCl 2 -treated poly-CdTe film measured at 80 K, similar to those used in CdTe solar cells, is shown in Fig. 2a . It features a shallow acceptor bound exciton peak [9] at 1.582 eV (783 nm) and a broad low-energy defect-related band centred at 1.42 eV (865 nm) that is typically observed in CdTe PL spectra. The low-energy band consists of a zero phonon line and multiple phonon replicas. The mass extracted from the diamagnetic shift of this band under applied magnetic fields up to 57T matches that of a free electron, indicating that the associated deep states are acceptors (see Supplementary Fig. S1 ). This assignment of a free electron to acceptor transition is consistent with previous reports [6] , [10] . Copper forms a neutral acceptor state (Cu Cd ) in CdTe with a binding energy of ~146 meV (ref. 6 ). It is a common impurity in CdTe source material and is also introduced into our sample within a thin Cu 1.4 Te adhesive layer between the glass/Mo substrate and poly-CdTe film. Secondary mass ion spectrometry measurements detect a constant Cu concentration of 10 19 cm −3 throughout the thickness of the poly-CdTe film. As similar spectra are observed in our as-grown poly-CdTe films (before CdCl 2 treatment), the Cu acceptor is probably the primary state involved in the low-energy transition. Chlorine introduced into the sample on CdCl 2 treatment may also form a deep acceptor A -centre complex with a nearest neighbour Cd vacancy and contribute to the low-energy PL as well [10] . Time-resolved PL (TRPL) measurements, displayed in Fig. 2b , indicate a fast radiative lifetime (~100 ps) for the bound excitons, which is consistent with other measurements in the literature [11] . However, the broad low-energy peak exhibits a much longer radiative lifetime (25 ns). This lifetime is similar to the low temperature decay times from bound N cluster states in dilute GaAs 1− x N x in which carriers trapped at deep states are forced to either radiatively recombine from the trap state or hop/tunnel to a nearby low-energy state [12] , [13] . 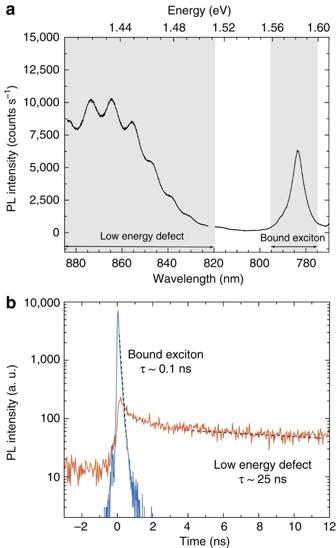Figure 2: Time-integrated and TRPL data. (a) Time-integrated spectrum of a CdCl2-treated poly-CdTe film measured at 80 K. (b) PL decay curves measured in the shaded portions of the spectrum inamarked low-energy defect (819–916 nm) and bound exciton (775–796 nm). Fits to the decay curves are shown as dashed black lines. Figure 2: Time-integrated and TRPL data. ( a ) Time-integrated spectrum of a CdCl 2 -treated poly-CdTe film measured at 80 K. ( b ) PL decay curves measured in the shaded portions of the spectrum in a marked low-energy defect (819–916 nm) and bound exciton (775–796 nm). Fits to the decay curves are shown as dashed black lines. Full size image PL images, presented in Fig. 3 , reveal an unusual inhomogeneous pattern of radiative recombination involving both bound excitons and deep acceptor states. Micron-scale markers were milled into the sample by a focused ion beam to correlate electron backscatter diffraction (EBSD) measurements of the grain structure with the PL images. The grain misorientation is shown in Fig. 3a , whereas the grain boundary positions are overlayed on the PL images in Fig. 3b–f for reference. Uniform excitation of PL across the entire image collection area with a defocused laser beam produced an irregular pattern of PL from all states, as presented in Fig. 3b . PL emitted only from bound excitons (782 nm, not shown) or deep acceptor states (865 nm, Fig. 3c ) exhibit similar patterns, but the bound exciton PL is weaker and more uniform. Neither of the PL patterns presented in Fig. 3b,c closely follow the exact grain arrangement measured by EBSD and suggest that the deep acceptors are unevenly dispersed throughout the film. Such inhomogenous distributions of low-energy luminescence have been observed by cathodoluminecence in poly-CdTe and have been widely reported in the literature [14] , [15] . Copper incorporation into the film as a result of both diffusion from the Cu 1.4 Te interlayer via fast diffusion channels and source material contamination during growth probably shapes the deep acceptor distribution. The post-growth anneal during CdCl 2 treatment may also provide an opportunity for Cu impurities to rearrange and aggregate within the film. 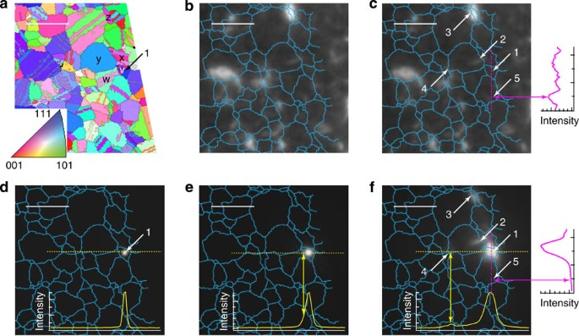Figure 3: PL images in a single location of a CdCl2treated poly-CdTe film. (a) EBSD image of the grain misorientation. The grain boundary positions are overlaid on the PL images inb–ffor reference. Images of PL at (b) all wavelengths and (c) 865 nm were obtained under widespread excitation with a defocused laser beam. The focused laser beam, shown indwas positioned in the grain marked ‘v’ ina. The corresponding images of PL at 783 and 865 nm are displayed ineandfrespectively. The inset indshows the profile of the reflected laser beam. The insets ineandfshow the PL intensity profiles along the horizontal dotted lines. The vertical yellow double arrow lines ineandfare used as guides to the eye to mark the same location between the dashed horizontal lines and the PL intensity profiles. The graphs at the far right display the PL intensity as a function of position along the dash-dotted vertical lines incandf. Explanations of the arrows are found in the text. Scale bars, 10 μm (upper left hand corners of the images ina–f). Figure 3: PL images in a single location of a CdCl 2 treated poly-CdTe film. ( a ) EBSD image of the grain misorientation. The grain boundary positions are overlaid on the PL images in b – f for reference. Images of PL at ( b ) all wavelengths and ( c ) 865 nm were obtained under widespread excitation with a defocused laser beam. The focused laser beam, shown in d was positioned in the grain marked ‘v’ in a . The corresponding images of PL at 783 and 865 nm are displayed in e and f respectively. The inset in d shows the profile of the reflected laser beam. The insets in e and f show the PL intensity profiles along the horizontal dotted lines. The vertical yellow double arrow lines in e and f are used as guides to the eye to mark the same location between the dashed horizontal lines and the PL intensity profiles. The graphs at the far right display the PL intensity as a function of position along the dash-dotted vertical lines in c and f . Explanations of the arrows are found in the text. Scale bars, 10 μm (upper left hand corners of the images in a – f ). Full size image PL images obtained under excitation with a focused laser beam (full width at half maximum~1 μm) depict the extent to which carriers diffuse through the poly-CdTe film. In the particular series of images presented here, the laser spot, displayed in Fig. 3d , is placed in the centre of the grain labelled ‘v’ in Fig. 3a , and its position is indicated by the arrow labelled ‘1’. On the basis of an absorption coefficient of 4 × 10 7 cm −1 at 515 nm (laser wavelength), the majority of photocarriers is expected to be generated within the first 150 nm of material around the laser spot, indicating that the effective diameter of photocarrier injection is about 300 nm greater than the laser beam width. The resulting bound exciton PL presented in Fig. 3e extends continuously over a few microns from the point of photocarrier injection. Intensity profiles measured through the centre of the reflected laser and emitted bound exciton PL spots along the displayed horizontal dotted lines are shown in the insets of Fig. 3d,e for comparison. The boundary between grains ‘v’ and ‘w’, indicated by the intersection of the dotted horizontal line and the solid double arrow vertical line in Fig. 3e , is located within the extent of the bound exciton PL spot, yet the intensity profile reveals no discontinuity that would indicate at least partial obstruction of exciton diffusion across the grain boundary. The results did not change when the position of the laser beam on the sample was shifted slightly in multiple directions, confirming that the measurement accurately portrays the benign behaviour of the grain boundary and does not result from a small error in the overlay of the EBSD and PL images. More remarkably, Fig. 3f shows that PL emanates from deep acceptor states (865 nm) at much greater distances (>10 μm) from the laser spot. This pattern includes a wide region of intense PL surrounding the point of photocarrier injection that continues into the grains labelled x, y and z as well as more distant regions corresponding to higher intensities of deep acceptor state PL in Fig. 3c . Arrows labelled ‘2’ and ‘3’ identify the most prominent regions emitting PL in Fig. 3c,f . Although less intense than regions 2 and 3, the region marked by the arrow ‘4’ also emits PL from deep defect states, as indicated by the peak in the intensity profile in the inset of Fig. 3f at the location of the double arrow vertical line. These images are representative of the PL behaviour observed over the entire sample (see Supplementary Figs S2 and S3 ) and from a larger set of CdCl 2 -treated poly-CdTe samples that was studied. Comparable time-integrated PL spectra, time-resolved decay curves and PL images were observed in as-grown poly-CdTe films as well. We emphasize here that the long-range PL from deep acceptor states is unlikely the result of photon recycling, in which the re-absorption of band edge PL leads to subsequent emission events. The absorption coefficient is very low for the sub-bandgap energy photons resulting from shallow bound exciton recombination, and absorption would occur over much longer-length scales than those observed for the deep acceptor state PL emission. The overall luminescence quantum efficiency of the deep acceptor states is also relatively low, and the resulting PL would be expected to be orders of magnitude weaker than the bound exciton PL. This is not the case here. PL of poly-GaAs A generalized model of carrier transport in polycrystalline materials was proposed by Seto [16] and later extended by Baccarani et al . [17] Carrier trapping by defects situated at grain boundaries leads to charge accumulation and the formation of a potential barrier that inhibits further charge transport across it [16] , [17] . This phenomenon has been widely studied in poly-GaAs, with measured barrier heights reaching 1 eV (refs 18 , 19 , 20 ). To place our results in the context of this wider body of work, PL imaging was also performed on large grained poly-GaAs wafers. The 80-K PL spectrum contains just a single excitonic peak at 820 nm, as expected. 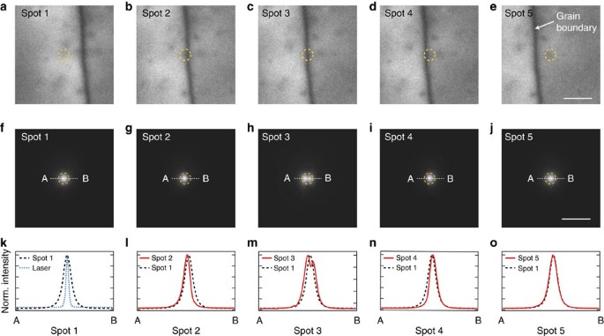Figure 4: PL images of a GaAs grain boundary. (a–e) PL images obtained at 820 nm under wide-area excitation with a defocused laser beam (spot size larger than the image) at five overlapping locations (spots 1–5 going froma–e). (f–j) PL images captured at the corresponding spots 1–5 obtained at 820 nm under excitation with a focused laser beam. The dotted circles mark the same positions in the defocused and focused excitation images. (k–o) Normalized PL intensity profiles along the horizontal dotted lines between positions A and B in images (f–j), respectively. The profile of spot 1 inkis repeated inl–ofor comparison. The profile of the laser beam size is also shown ink. Scale bars, 10 μm (lower right-hand corners of images (e,j), which correspond to all of the images. Figure 4a–e shows a series of PL images of a single-grain boundary obtained under wide-area excitation with a defocused laser beam. The boundary manifests as a line of high non-radiative recombination. Figure 4f–j shows the corresponding PL images captured as a focused laser beam was scanned across the boundary. Photocarrier injection away from the grain boundary ( Fig. 4f,j ) results in a radially uniform PL spot with a Gaussian intensity decay ( Fig. 4k,o ). However, PL is curtailed in the direction of the grain boundary when the laser is placed in its immediate vicinity ( Fig. 4g,i ), and PL is not observed in the adjacent grain or at any remote locations. The preferential decrease in PL at the grain boundary is most evident by comparing the intensity profiles of spot 1 with spots 2 and 4 in Fig. 4l,n . In fact, a high degree of non-radiative recombination at the grain boundary is observed under direct photocarrier injection, as shown in Fig. 4h . A similar reduction in PL intensity near the grain boundaries is not observed in the CdTe samples. Figure 4: PL images of a GaAs grain boundary. ( a – e ) PL images obtained at 820 nm under wide-area excitation with a defocused laser beam (spot size larger than the image) at five overlapping locations (spots 1–5 going from a – e ). ( f – j ) PL images captured at the corresponding spots 1–5 obtained at 820 nm under excitation with a focused laser beam. The dotted circles mark the same positions in the defocused and focused excitation images. ( k – o ) Normalized PL intensity profiles along the horizontal dotted lines between positions A and B in images ( f – j ), respectively. The profile of spot 1 in k is repeated in l – o for comparison. The profile of the laser beam size is also shown in k . Scale bars, 10 μm (lower right-hand corners of images ( e , j ), which correspond to all of the images. Full size image Compared with GaAs, grain boundaries in CdCl 2 -treated poly-CdTe do not appear to significantly inhibit exciton diffusion or act as sites of substantial non-radiative recombination. A number of studies published in the literature provide evidence that the potential barriers at grain boundaries at room temperature actually help to separate majority and minority carriers and aid the transport of minority carriers to the junction [2] , [21] . At lower temperatures, however, this barrier to majority carriers is expected to be smaller, perhaps on the order of 10–20 meV, which would explain their relative transparency to exciton diffusion at 80 K (refs 21 , 22 ). Carrier trapping by the high densities of deep acceptor states in the surrounding bulk grain material may also act to lower the potential barrier by screening the charge accumulation at the grain boundary [23] . Carrier hopping in poly-CdTe The large separation between the points of photocarrier injection and PL emission from deep acceptor states, in contrast to that of the bound exciton, suggests that the deep acceptor states mediate hole diffusion over long distances. The long lifetimes measured by TRPL are consistent with trapping behaviour, in which carriers can either jump from one trap state to another or radiatively recombine [13] . Carrier transport through these states therefore necessarily requires that they form percolated networks that support hopping conduction. Evidence of variable range hopping in both poly-CdTe and Cu(In,Ga)Se 2 materials has been detected via electrical measurements, which reveals a large drop in the conductivity and mobility at lower temperatures and a transition to a regime that follows a exp( T −1/4 ) behaviour [24] , [25] , [26] , [27] , [28] . Hall measurements are often difficult to perform on p -type poly-CdTe films because of their low free-carrier concentrations and mobility. To probe the trap state behaviour in our material, admittance spectroscopy (AS) was carried out on completed poly-CdTe devices with comparable Cu concentrations [29] . Differential capacitance spectra as a function of temperature yield a hole trap activation energy of 152 meV, which is consistent with the acceptor-binding energy determined from the PL measurements. Mobility values extracted from bias-dependent dielectric relaxation measurements were found to drop by an order of magnitude between 300 K (0.95 cm 2 V −1 s −1 ) and 100 K (7.1 × 10 −2 cm 2 V −1 s −1 ). At low temperatures, a transition between two transport regimes is marked by the change in the slope of the μ versus T trend near 80 K in Fig. 5 . Similar deviations in the μ versus T data of poly-Cu(In,Ga)Se 2 material have been linked to a shift to variable range hopping in an impurity band [25] . Without additional data points and precise temperature-dependent carrier concentration data, it is difficult to accurately determine the power dependence of the data at the lower end of this temperature range. We also note that it is very probable that several transport mechanisms operate simultaneously in this regime. However, the experimental transport data suggest that variable range hopping occurs in our poly-CdTe material at low temperatures. The fact that it is observed up to 80 K is a consequence of the relatively large acceptor-binding energy. 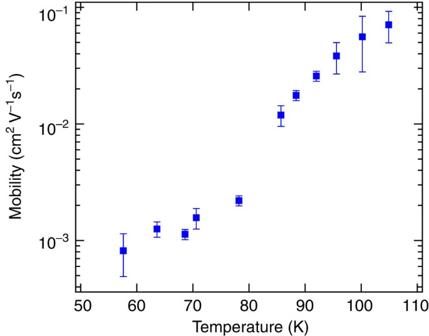Figure 5: Mobility versus temperature. The hole mobility values were extracted from bias-dependent AS measurements. The change in theμversusTtrend near 80 K suggests a transition to hopping-dominated transport. The error bars represent one s.d. of uncertainty estimated from linear fitting of the bias-dependent AS data when extracting the hole mobility. Figure 5: Mobility versus temperature. The hole mobility values were extracted from bias-dependent AS measurements. The change in the μ versus T trend near 80 K suggests a transition to hopping-dominated transport. The error bars represent one s.d. of uncertainty estimated from linear fitting of the bias-dependent AS data when extracting the hole mobility. Full size image Physically, the deep acceptor states can support variable range hopping conduction of holes without activation into the valence band if they are present in high enough concentrations that the wavefunction of a hole localized on one acceptor overlaps neighbouring acceptors. The Mott criterion for impurity band formation therefore requires that the deep acceptor states be spaced on average a ≤3 a 0 , where a 0 is the Bohr radius of the carrier, , and N trap is the trap concentration [28] . Assuming a dielectric constant of ε r =10.6 and a hole mass of m* / m 0 =0.6, the hole Bohr radius is roughly 10 Å in CdTe, and a trap density of N trap =10 18 cm −3 would yield an average intertrap spacing of a =70 Å. Further considering that the density of Cu impurities in the poly-CdTe films is ~10 19 cm −3 and that they are inhomogenously distributed, it is probable that the required conditions for impurity band formation are met within certain high-concentration regions or connecting channels. This picture of impurity band conduction is supported by previous studies that link higher Cu concentrations near grain boundaries with higher conductivity [30] . Selective redistribution of photogenerated holes through a network of deep acceptor state impurity band channels is experimentally corroborated on comparing the PL patterns generated by wide area uniform and focused excitation presented in Fig. 3c,f , respectively. Some regions of elevated deep acceptor densities that emit strong PL under wide-area excitation (notably 3 and 4 in Fig. 3c,f ) continue to luminesce when carriers are photogenerated >10 μm away in grain ‘v’ under focused excitation. In these cases, percolated networks of defect states probably form pathways for hole diffusion, although the pathways themselves may not have high enough deep acceptor densities to support intense radiative recombination. Other regions of the film, however, appear to lack such a network. Region 5 emits measurable PL under wide-area excitation, indicated by the peak in the intensity profile measured along the vertical dash-dotted line in Fig. 3c . Yet, when photocarriers are selectively injected into grain ‘v’ at location 1, no significant PL emission is observed at 5, as indicated in the intensity profile measured along the corresponding vertical dash-dotted line in Fig. 3f . The selective population of and radiative recombination from deep acceptor states remotely located within a common radius from a focused point of photocarrier injection thus provide evidence of defect network-mediated hole transport. Grain boundaries may also facilitate carrier diffusion, as suggested by several previous studies [2] , [21] , [30] ; however, the resolution of the PL imaging technique precludes categorical determination of this effect. Nevertheless, the high PL intensities from regions located in the grain interiors clearly demonstrate that this is not a necessary condition for long-range hole transport (see Fig. 3 and Supplementary Fig. S3 ). It should be noted that the deep acceptor PL and hence network-mediated hole diffusion are observed only at low temperatures. The longest distance that PL is detected from the point of carrier generation (>10 μm) is also not representative of the average diffusion length in the material, as most of the PL is generated much closer to the photoinjection point. Although the PL imaging technique presented here only probes the distance of hole diffusion that ends in radiative recombination, carrier capture at non-radiative recombination sites also affects transport in the material. As evidenced by the hopping behaviour determined from the low-temperature AS measurements, holes are expected to primarily hop between the deep acceptor states that make up the impurity band until they radiatively recombine or encounter an even deeper non-radiative state [13] . This picture is consistent with the long radiative lifetimes measured that give carriers enough time to hop between several sites. Experimental methods combining spatially localized carrier injection and electrically detected current mapping must be developed to probe the relative influence of radiative and non-radiative recombination sites on long-range carrier transport. However, the measurements presented here demonstrate the existence of long-range hole diffusion through deep trap states. From a broader perspective, these results have implications to further the general understanding of impurity band transport. Percolation phenomena in semiconductor systems are of considerable interest, especially those that are assumed to be inhomogeneous. The ability to directly observe the spatial distribution of carrier diffusion from a single point of photoinjection provides important insight into the relationships between microstructure, impurity state distribution and carrier transport mechanisms. In the present case of poly-CdTe, conservation of the spatial correlation between carrier generation and recombination reveals new information about the role that non-uniform distribution of impurity states has in the conduction of carriers at low temperatures. This technique also offers a new avenue for investigating spatially and energetically inhomogenous carrier transport in a wide range of other polycrystalline material systems. Material preparation P-type poly-CdTe films (6 μm thick) were grown by close space sublimation (CSS) at 600 °C on a 10-nm Cu 1.4 Te/Mo/glass substrate. Post-growth CdCl 2 treatment was performed at 450 °C by CSS. The samples were polished to prevent significant laser scatter, and the resulting damage was removed with a 0.5% Br:methanol etch. PL measurements of poly-GaAs were performed on polished semi-insulating GaAs wafers with large (>1 mm) grains. AS measurements were performed on fully processed poly-CdTe solar cell devices. The device layer stack consisted of Corning 7059 glass, 400 nm SnO 2 :F, 100 nm SnO 2 , 100 nm CdS grown by chemical-bath deposition at 92 °C, 5 μm CdTe grown by CSS at 620 °C and 500 nm of ZnTe:Cu (2% weight Cu) grown by radio frequency magnetron sputtering in 10 mTorr Ar at 300 °C. Following deposition, a CdCl 2 treatment was applied at 400 °C in O 2 /He for 5 min. A 90-nm ITO layer and a 50-nm Ni/3 μm Al metal grid were then added as a back contact. Microstructural analysis EBSD analysis was performed in a field emission gun scanning electron microscope Nova 630 NanoSEM from FEI, using an EDAX Pegasus/Kikari A40 system. Optical spectroscopy Time-integrated and TRPL measurements were performed with a mode-locked Ti:sapphire laser set at a wavelength of 763 nm, a power density of 0.5 μJ cm −2 and a 2-MHz repetition rate. The PL signal was detected with a photon-counting streak camera. PL imaging measurements were carried out with a 515-nm cw laser. The incident focused laser intensity on the sample was varied between 10 2 –10 4 W cm −2 (2–200 μW total power) to excite sufficient PL intensities for detection. The emission pattern did not change with changing laser intensity. PL was collected with a × 50 objective lens and was focused onto an Andor CCD camera with 16 μm pixels. The spatial resolution of the system is ~0.9 μm. All measurements were performed at 80 K. Magneto-PL measurements were carried out in a 60-T-long pulse magnet using a solid-state laser (515 nm, 1 W cm −2 ) to excite PL through a 550-μm-diameter optical fibre coupled to the sample. The spectra were measured at 1.6 K. Admittance spectroscopy AS was performed with an Agilent 4294A impedence analyser with direct current bias varied from −1.2 to +0.7 V. The frequency and temperature were varied from 10 3 to 10 8 Hz and from 50 to 300 K, respectively. The carrier mobility measurement exploits the bias dependence of the ‘modified’ dielectric relaxation frequency in a semiconductor in the presence of a depletion region. Any neutral semiconductor with carrier density N and mobility μ exhibits dielectric relaxation at an intrinsic frequency ω dr =σ/ε where σ=qNμ is the conductivity and ε is the permittivity. If part of the semiconductor is depleted and the rest remains neutral, as is the case in a solar cell, then the ‘modified’ dielectric relaxation frequency becomes ω mdr = ω dr ( W / t ), where W is the depletion region width and t is the total thickness of the semiconductor. The equivalent circuit consists of the series connection of the depletion capacitance (representing the contribution from the depletion region) and the bulk conductance and capacitance connected in parallel (representing the contribution from the neutral region). AS is used to identify ω mdr by observing that the measured capacitance below and above ω mdr are that of the depletion region, that is, ε / W , and the geometrical capacitance (that is, ε / t ), respectively. As the depletion width W varies with bias V , the ‘modified’ dielectric relaxation frequency also depends on V according to: where V bi is the built-in voltage associated with the depletion region. From the slope of versus V , one can extract the mobility according to: where the carrier density N is determined from capacitance–voltage measurement and the thickness of the semiconductor t is determined by depth profiling measurement. How to cite this article: Alberi, K. et al . Measuring long -range carrier diffusion across multiple grains in polycrystalline semiconductors by photoluminescence imaging. Nat. Commun. 4:2699 doi: 10.1038/ncomms3699 (2013).